eEF2 and Ras-GAP SH3 domain-binding protein (G3BP1) modulate stress granule assembly during HIV-1 infection Stress granules (SG) are translationally silent sites of RNA triage induced by environmental stresses including viral infection. Here we show that HIV-1 Gag blocks SG assembly irrespective of eIF2α phosphorylation and even when SG assembly is forced by overexpression of Ras-GAP SH3 domain-binding protein (G3BP1) or TIAR. The overexposed loops in the amino-terminal capsid domain of Gag and host eukaryotic elongation factor 2 (eEF2) are found to be critical for the SG blockade via interaction. Moreover, cyclophilin A (CypA) stabilizes the Gag–eEF2 association. eEF2 depletion not only lifts the SG blockade but also results in impaired virus production and infectivity. Gag also disassembles preformed SGs by recruiting G3BP1, thereby displacing eEF2, revealing another unsuspected virus–host interaction involved in the HIV-1-imposed SG blockade. Understanding how HIV-1 counters anti-viral stress responses will lay the groundwork for new therapeutic strategies to bolster host cell immune defences against HIV-1 and other pathogens. Following viral infection, host cells respond by mounting robust, anti-viral immune responses to create an unfavourable environment for viral replication [1] . A central feature of the cellular stress response is the reprogramming of host cell mRNA translation and subsequent induction of stress granules (SGs) [2] . SGs are translationally silent ribonucleoprotein complexes (RNPs) that assemble during various types of cellular stresses including viral infection, physical and environmental trauma [3] . These contain heterogeneous mRNAs and translation factors, including eIF4G, eIF4E, eIF3, eIF2 and PABP and other RNA-binding proteins including TIA-1, TIA-1-related RNA-binding protein (TIAR), Ras-GAP SH3 domain-binding protein (G3BP1) and Staufen1 (refs 1 , 3 ). SGs cycle through phases of assembly, persistence or disassembly [4] , [5] . Although a genome-wide RNA interference (RNAi) screen identified factors that impact SG assembly [6] , the molecular mechanisms by which SG assembly is initiated have not been fully elucidated. However, it has been determined that initial SG assembly requires aggregation of SG-dependency factors (SGDFs), including G3BP1 (ref. 7 ) or TIA-1/TIAR [8] . Nevertheless, two recent studies have shown that SGs could be disassembled due to the reactivation of mTORC1 (ref. 9 ) or cleared via autophagy [10] . Human immunodeficiency virus type 1 (HIV-1) is the etiologic agent of acquired immunodeficiency syndrome (AIDS) [11] . We previously unveiled the ability of HIV-1 to block SG assembly in cells exposed to sodium arsenite (Ars) and found that the genomic viral RNA (vRNA) and Gag polyprotein localized to Staufen1-containing RNPs [12] . Here we show that under transient expression or infection, HIV-1 blocks SG assembly in an eIF2α phosphorylation (eIF2α-P) independent manner in cells exposed to pateamine A (PatA) or in cells overexpressing G3BP1/TIAR. Moreover, we show that the capsid (CA) domain of Gag elicits a blockade to SG assembly via an interaction with the eukaryotic elongation factor (eEF) and SGDF, eEF2 that is stabilized by a Gag–cyclophilin A (CypA) association. The SG blockade is reversed on eEF2 depletion, which also negatively impacts on virus production and infectivity. We find that mutations in the surface-exposed loops of the N-terminal domain of CA fail to block SG assembly under stress conditions. Furthermore, Gag disassembled preformed SGs via an interaction with G3BP1. This work describes novel countermeasures elicited by the HIV-1 Gag protein to remodel cellular RNPs during cellular stress. HIV-1 impairs SG assembly independent of eIF2α-P The phosphorylation of eIF2α is the most universal response to stress that leads to the rapid assembly of SGs [13] . eIF2α-P subsequently associates with eIF2B resulting in the inhibition of GDP–GTP exchange, thereby compromising the translation ternary complex [14] . SG assembly also occurs by G3BP1 or TIAR overexpression [3] as well as in eIF2α-P-independent manner by PatA, which hyperactivates the eIF4A helicase to inhibit translation initiation by disrupting the eIF4F complex [15] . We have previously shown that HIV-1 blocks SG assembly but did not modulate eIF2α-P levels [12] . To determine whether or not the HIV-1-mediated blockade to SG assembly was independent of eIF2α-P, the localization of the SG markers G3BP1 and TIAR was determined by immunofluorescence (IF) and laser scanning confocal microscopy in both human HeLa and Jurkat T cells treated with PatA. HeLa and Jurkat T cells ( Fig. 1a,c , respectively) were transfected with the infectious HIV-1 molecular clone pNL4-3 and after 48 h and 6 days post transfection, respectively, cells were exposed to PatA and Ars. In mock-transfected HeLa and Jurkat T-cell lines, treatment with either PatA or Ars induced abundant SG assembly in >95% of cells ( Fig. 1a,c , yellow arrows; Fig. 1b,d , grey bar), while HIV-1-expressing cells imposed a strong block to SG assembly in both cell types ( Fig. 1a,c , red arrows; Fig. 1b,d , black bar: HeLa: PatA: 9.5%; Ars: 9.4%; Jurkat T: PatA: 16%; Ars: 20%). PatA treatment did not increase eIF2α-P levels compared with that of cells treated with Ars alone ( Fig. 1b,d , compare lanes 2 and 3). Furthermore, HIV-1 expression did not alter eIF2α-P in Ars-treated cells ( Fig. 1b,d , compare lanes 3 and 6) in agreement with our earlier work [12] . In a tandem approach, we overexpressed G3BP1 or TIAR to induce the spontaneous assembly of SGs. Surprisingly, HIV-1 blocked SG assembly in these conditions ( Fig. 1e ). G3BP1 or TIAR overexpression had no effect on eIF2α-P or HIV-1 expression ( Fig. 1f ). Finally, to examine whether or not the SG blockade is a general feature of HIV-1 infection in ex vivo CD4+ T cells, we isolated T cells from treatment-naive individuals with distinct disease courses: a long-term nonprogressor (LTNP; Fig. 1g ) and a chronically infected progressor ( Fig. 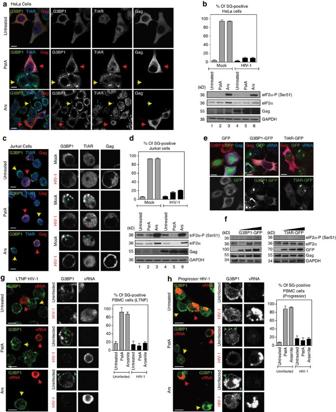Figure 1: HIV-1 blocks SG assembly irrespective of eIF2α-P. HeLa (a) and Jurkat cells (c) were transfected with HIV-1 pNL4-3 and were exposed to PatA (middle panel) for 1 h or sodium Ars (bottom panel) for 45 min. Cells were stained for G3BP1, TIAR and Gag. Yellow arrows: mock-transfected cells. Red arrows: HIV-1-expressing cells. Scale bar, 10 μm. Magnifications of cells (c) on right show presence of SG indicated with green arrows. (b,d) Top: quantification of SG in mock-transfected (grey bars) or HIV-1 expressing (black bars) cells froma,c. Data are presented as mean±s.d. from three separate experiments with at least 100 cells each analysed. Bottom: cell lysates were analysed for eIF2α-p (Ser51), eIF2α, Gag and GAPDH. (e) HeLa cells expressing HIV-1 and G3BP1-GFP or TIA-1-GFP (0.5–2 μg) were processed for FISH/IF analyses and stained for Gag and vRNA. Scale bar, 10 μm. (f) Immunoblot analysis of whole-cell lysate fromeis shown. (g,h) PBMCs from two HIV-1-infected subjects with different disease outcomes were subjected to stress and analysed by FISH/IF. Cells from long-term nonprogressor (LTNP;g) and typical progressor (h) were fixed and stained for G3BP1 and vRNA. Scale bar, 5 μm. Magnifications of cells on right show presence of SG indicated with green arrows. Right Panel: quantification of SG in uninfected (grey bars) or HIV-1-infected (black bars) cells fromg,h. Data are presented as mean±s.d. from three separate experiments with at least 50 cells each analysed. 1h ; Supplementary Table 1 ). Peripheral blood mononucleated cell (PBMCs) were exposed to stress as described in Methods. Endogenous G3BP1 staining was used to measure the ability of cells to induce SGs. There was no evidence of SGs in patients’ cells expressing HIV-1 ( Fig. 1g,h , red arrows; graphs, black bar: LTNP: PatA: 11.25%; Ars: 17.7%; progressor: PatA: 12.2%; Ars: 15.75%) suggesting that the ability of HIV-1 to block SG assembly does not depend on the course of HIV-1 progression. Figure 1: HIV-1 blocks SG assembly irrespective of eIF2α-P. HeLa ( a ) and Jurkat cells ( c ) were transfected with HIV-1 pNL4-3 and were exposed to PatA (middle panel) for 1 h or sodium Ars (bottom panel) for 45 min. Cells were stained for G3BP1, TIAR and Gag. Yellow arrows: mock-transfected cells. Red arrows: HIV-1-expressing cells. Scale bar, 10 μm. Magnifications of cells ( c ) on right show presence of SG indicated with green arrows. ( b , d ) Top: quantification of SG in mock-transfected (grey bars) or HIV-1 expressing (black bars) cells from a , c . Data are presented as mean±s.d. from three separate experiments with at least 100 cells each analysed. Bottom: cell lysates were analysed for eIF2α-p (Ser51), eIF2α, Gag and GAPDH. ( e ) HeLa cells expressing HIV-1 and G3BP1-GFP or TIA-1-GFP (0.5–2 μg) were processed for FISH/IF analyses and stained for Gag and vRNA. Scale bar, 10 μm. ( f ) Immunoblot analysis of whole-cell lysate from e is shown. ( g , h ) PBMCs from two HIV-1-infected subjects with different disease outcomes were subjected to stress and analysed by FISH/IF. Cells from long-term nonprogressor (LTNP; g ) and typical progressor ( h ) were fixed and stained for G3BP1 and vRNA. Scale bar, 5 μm. Magnifications of cells on right show presence of SG indicated with green arrows. Right Panel: quantification of SG in uninfected (grey bars) or HIV-1-infected (black bars) cells from g , h . Data are presented as mean±s.d. from three separate experiments with at least 50 cells each analysed. Full size image HIV-1-specific SG assembly blockade Retroviruses can be classified into those that have simple genomes (α and γ retroviruses) and those with complex genomes (lentiviruses and deltaviruses; Fig. 2a ). To assess the ability of other retroviruses to affect SG assembly, we transfected HeLa cells with either HIV-2, simian immunodeficiency virus (SIV), feline immunodeficiency virus (FIV), murine leukemia virus (MLV) and Rous sarcoma virus (RSV) proviral DNA and exposed these cells to PatA to induce SGs. For equine infectious anemia virus (EIAV), we produced VSVg-pseudotype particles with green fluorescent protein (GFP) and HeLa cells infected. None were able to block SG assembly as did HIV-1 with >70% of retrovirus-expressing cells exhibiting SG ( Fig. 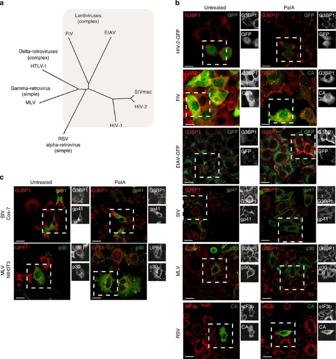Figure 2: The ability to block stress is not innate to all retroviruses. (a) Phylogenetic tree of major retrovirus families used in this study (envgene). (b) HeLa cells were transfected or infected with HIV-2, SIV, EIAV, FIV, MLV or RSV and 48 h later were exposed to PatA. Cells were stained for gp41(SIV), p30(MLV), CA(FIV/RSV), G3BP1 and eIF3b, as indicated. Squares represent regions of interest. Scale bar, 30 μm. (c) NIH3T3 cells were transfected with MLV DNA (top) or Cos-7 cells were transfected with SIV DNA (bottom) and at 48 h exposed to PatA. Cells were stained for gp41(SIV), G3BP1, p30 (MLV) and UPF-1 as indicated. Scale bar, 30 μm. 2b ; Supplementary Table 2 ). Furthermore, PatA-treated mouse NIH3T3 cells transfected with MLV or monkey Cos-7 cells transfected with SIV exhibited robust SG assembly ( Fig. 2c ) when compared to the abundance of SGs in HIV-1-expressing Jurkat T cells ( Fig. 1c ). While Legros et al . [16] showed that HTLV-1 is able to inhibit SG assembly, none of the other retroviruses tested had this capacity. Figure 2: The ability to block stress is not innate to all retroviruses. ( a ) Phylogenetic tree of major retrovirus families used in this study ( env gene). ( b ) HeLa cells were transfected or infected with HIV-2, SIV, EIAV, FIV, MLV or RSV and 48 h later were exposed to PatA. Cells were stained for gp41(SIV), p30(MLV), CA(FIV/RSV), G3BP1 and eIF3b, as indicated. Squares represent regions of interest. Scale bar, 30 μm. ( c ) NIH3T3 cells were transfected with MLV DNA (top) or Cos-7 cells were transfected with SIV DNA (bottom) and at 48 h exposed to PatA. Cells were stained for gp41(SIV), G3BP1, p30 (MLV) and UPF-1 as indicated. Scale bar, 30 μm. Full size image Gag inhibits SG assembly Several studies have established that the assembly/disassembly of SGs can be influenced by viral proteins (reviewed in ref. 17 ). To elucidate the molecular mechanisms by which HIV-1 inhibits SG assembly, we attempted to map the viral determinant in HIV-1 that mediates SG inhibition. We first transfected HeLa cells with a battery of HIV-1 proviral constructs based on pNL4-3, a provirus that expresses the full complement of viral proteins ( Fig. 3a ; Supplementary Fig. 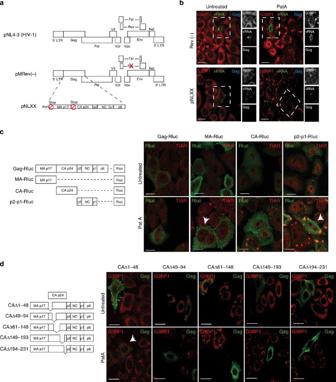Figure 3: Gag elicits the SG assembly blockade. (a) Organization of the HIV-1 viral proteins in the genome is shown, as well as proviral deletion mutants lacking Gag, pMRev(−) and pNLXX. (b) HeLa cells were transfected with pMRev(−) or pNLXX proviral deletion mutants, then exposed to PatA. Cells were stained for G3BP1, vRNA and Gag. Squares represent regions of interest. Scale bar, 20 μm. (c) HeLa cells were transfected with different plasmids expressing Gag and deletion mutants fused to Rluc and exposed to PatA. Cells were stained for Rluc and TIAR as indicated. Scale bar, 10 μm. (d) HeLa cells were transfected with five CA-deletion mutants and exposed to PatA. Cells were stained for G3BP1 and Gag (p17). Scale bar, 15 μm. White arrows identify Gag mutants unable to prevent the SG assembly. 1 ; and listed in Supplementary Table 3 ), and at 48 h exposed cells to PatA. By combined fluorescence in situ hybridization/IF (FISH/IF) co-analyses, we visualized the distribution of vRNA and/or Gag to identify HIV-1(+) cells and that of SGs exhibited by large G3BP1 foci. pNL4-3 proviral constructs harbouring individual gene deletions in vif , vpr , vpu , env and nef led to complete SG inhibition in cells exposed to PatA ( Supplementary Table 3 ; ref. 18 ). Additional proviral constructs, with various genetic backgrounds, encoding additional specific mutations were subsequently tested, including proviruses with mutations in the Gag-myristoylation signal (mediating membrane association) and p6 Gag domain (mediating interactions with the endosomal sorting complexes required for transport (ESCRT) machinery for virus budding; listed in Supplementary Table 3 ). The use of these proviruses, although defective in multiple viral genes, was possible since each viral gene was ruled out as a putative SG effector. Since HTLV-1 Tax protein inhibits the assembly of SGs [16] , we excluded the role of HIV-1 Tat with the use of the proviral construct, pTat(−)GV/4GS, which contains a deletion of the tat gene, but achieves HIV-1 expression by long terminal repeat region (LTR) transactivation via Gal4-VP16, as described in Methods (listed in Supplementary Table 3 ). In contrast, HIV-1 failed to prevent SG assembly when the proviral construct that harbours a mutation in rev was expressed (pMRev(−); Fig. 3b ; Supplementary Table 3 ). Failure to express Rev has no effect on HIV-1 transcription but leads to a block in nuclear export of the unspliced vRNA and the singly spliced vpr and vpu mRNAs. As Vpr and Vpu were not responsible for the SG blockade, nor were any of the pol genes (using Gag/Pol vector lacking the viral protease (PR), pVRC4000 PR− and pVRC4200 PR+, listed in Supplementary Table 3 ), we turned our attention to Gag because its synthesis would be abrogated in Rev(−) conditions. To corroborate these findings, the pNL4-3-based proviral DNA, pNLXX, which contains two stop codons in the Gag-coding region, was expressed ( Fig. 3a ) [19] . This construct failed to block SG assembly in >95% of Gag-expressing cells (pNLXX; Fig. 3b ; Supplementary Table 3 ). Since these results strongly suggested that Gag was responsible for preventing SG assembly, we confirmed that cells expressing Gag alone and that were subjected to stress did not assemble SGs (Gag-Rluc; Fig. 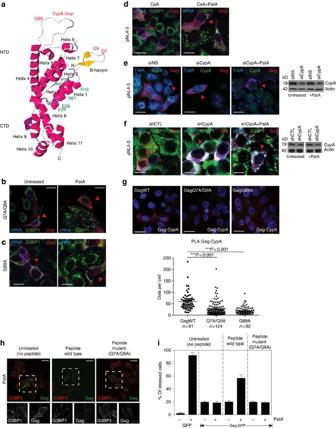Figure 4: Overexposed surface loops in NTD of CA play a crucial role in the inhibition of SG assembly. (a) Location of CA amino-acid residues conferring SG dependency are shown in red on the structural model of CA monomer extracted from the hexameric structure (PDB: 3H4E). CA substitutions that did not alter the ability to block SG assembly are shown in green. (b) HeLa cells were transfected with five NTD point mutants of CA and exposed to PatA (here Q7A/Q9A). Cells were stained for vRNA, G3BP1 and Gag (p17). Scale bar, 15 μm. (c) HeLa cells were transfected with G89A CA mutant or (d) WT (pNL4-3) HIV-1 provirus. After 12 h, cells were incubated with 2.5 μM of CsA for 8 h and exposed to PatA. Cells were fixed and stained for vRNA, G3BP1 and Gag (p24). Scale bar, 15 μm. Hela cells were treated with siCypA (e) or shCypA (f), transfected with WT (pNL4-3) HIV-1 provirus and exposed to PatA. Cells were fixed and stained for G3BP1, TIAR, CypA, vRNA and Gag (p24), as indicated. Scale bar, 10 μm. Red arrows indicate HIV-1-expressing cells. Immunoblot analysis of whole-cell lysates frome,fare shown in right panels. (g) Top: CA mutants fail to bind CypAin situ. Nuclei were stained with DAPI (blue), and PLA was performed for Gag and CypA association (red). Bottom: relative quantitation representing spots per cell. Data are represented as mean±s.e.m. Statistical analysis was performed with a one-way analysis of variance (ANOVA) combined with the Bonferroni’s post test. (h) Hela cells expressing Gag-GFP were treated with a WT or Q7A/Q9A peptide for 1 h and subjected to PatA. Cells were stained for G3BP1. Scale bar, 15 μm. (i) SG present in cells fromhwere quantified.n=100 cells from three separate experiments. Data are represented as mean±s.d. 3c ; Supplementary Table 4 ). Given that Gag is a polyprotein cleaved by viral PR into the subdomains, matrix (MA/p17), apsid (CA/p24), p2, nucleocapsid (NC/p7), p1 and p6, we mapped the Gag domain involved in the block to SG assembly. Three deletion mutants containing different Gag subdomains (MA, CA and p2-p1) fused in-frame to Renilla luciferase (Rluc) previously described by our laboratory [20] ( Fig. 3c ), as well as the MA-deleted mini-Gag proviruses [21] were utilized ( Supplementary Fig. 1 ; Supplementary Table 4 ). IF analyses confirmed that Gag mutants lacking CA could not suppress SG in >70% of transfected cells subjected to PatA ( Fig. 3c ; Supplementary Table 4 ). These results indicate that the CA/p24 domain is sufficient to mediate the SG blockade. CA/p24 contains two structural domains, the N-terminal assembly domain (NTD) and the carboxy-terminal dimerization domain. The NTD is composed of seven α-helices and an N-terminal β-hairpin [22] , while the carboxy-terminal dimerization domain is composed of four α-helices [23] . To assess which domain of CA/p24 participates in the block to SG assembly, five deletion mutants in CA/p24 were designed to progressively eliminate resolved three-dimensional (3D) structures [24] ( Fig. 3d ). The deletion mutant of the β-hairpin and helices 1 and 2 in the N terminus of CA (CAΔ1-48) was the only mutant that lost the ability to block SG assembly with >85% of cells exhibiting SG ( Fig. 3d ; Supplementary Table 4 ). Figure 3: Gag elicits the SG assembly blockade. ( a ) Organization of the HIV-1 viral proteins in the genome is shown, as well as proviral deletion mutants lacking Gag, pMRev(−) and pNLXX. ( b ) HeLa cells were transfected with pMRev(−) or pNLXX proviral deletion mutants, then exposed to PatA. Cells were stained for G3BP1, vRNA and Gag. Squares represent regions of interest. Scale bar, 20 μm. ( c ) HeLa cells were transfected with different plasmids expressing Gag and deletion mutants fused to Rluc and exposed to PatA. Cells were stained for Rluc and TIAR as indicated. Scale bar, 10 μm. ( d ) HeLa cells were transfected with five CA-deletion mutants and exposed to PatA. Cells were stained for G3BP1 and Gag (p17). Scale bar, 15 μm. White arrows identify Gag mutants unable to prevent the SG assembly. Full size image NTD of CA plays a crucial role in the SG assembly The NTD of CA domain contains several mutations that have been previously characterized [25] . We chose five of these mutants (Q7A/Q9A, R18A/N21A, E28A/E29A, P38A and A42D) that have different phenotypic characteristics ( Fig. 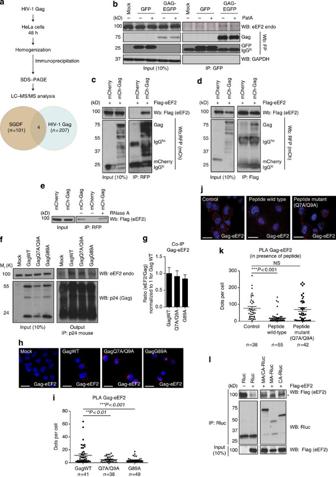Figure 5: Gag interacts with eEF2. (a) Flowchart of the proteomics analyses used to define Gag-binding proteins (top). Venn diagram exhibiting the number of overlapping hits between Gag-binding partners with SGDFs (bottom)6. (b) HeLa cells were transfected with 5 μg of Gag-EGFP or GFP alone and 48 h later were exposed to PatA, lysed and cell extracts were subjected to IP with an anti-GFP antibody. The presence of endogenous eEF2 in the immunoprecipitates was assessed by western blotting. Ten per cent of total cell lysates used in IP are shown as input. (c,d) HEK293T cells were co-transfected with mCherry or mCh-Gag and Flag-eEF2 and collected for IP with (c) anti-RFP (to detectmCherry) or (d) anti-Flag followed with immunoblot analysis. (e) Cell lysates were incubated in the presence (+) or absence (−) of RNase A for 30 min before IP analysis. Data shown are representative of three experiments. (f) HeLa cells were transfected with HIV-1 WT (pNL4-3) or CA mutants’ (Q7A/Q9A, G89A) provirus and collected for IP with anti-p24 (to detectGag). (g) Relative quantitation of eEF2 co-IP with Gag. Ratio of eEF2/Gag forn=3 experiments. Data are normalized to 1 for Gag WT and represented as mean±s.d. (h) Cells fromfwere subjected to PLA. Nuclei stained with DAPI (blue); PLA performed for Gag and eEF2 (red). Scale bar, 15 μm. (i) Relative quantitation of Gag–eEF2 association. Spots per cell were counted. Data represented as mean±s.e.m. of three independent experiments. Statistical analysis was performed with a one-way ANOVA combined with the Bonferroni’s post test. (j) HIV-1-expressing HeLa cells were treated with a WT or Q7A/Q9A peptide for 1 h and subjected to PatA. PLA was performed. Top panel: nuclei stained with DAPI (blue); PLA performed for Gag and eEF2 (red). Scale bar, 15 μm. (k) Relative quantitation of Gag–eEF2 association. Spots per cell were counted. Data are represented as mean±s.e.m. of three independent experiments. Statistical analysis was performed with a one-way ANOVA combined with the Bonferroni’s post test. (l) HEK293T cells were co-transfected with Gag-deletion mutants (MA/CA; MA; CA) fused to Rluc and Flag-eEF2. Cell lysates were IP with anti-RLuc and immunoblotted with anti-Flag (*nonspecific band). 4a ; Supplementary Table 5 ). Q7A/Q9A was the only proviral CA mutant that failed to repress the stress response (in 72% of the cells; Fig. 4b ), whereas the other four CA proviral mutants retained the SG inhibition (listed in Supplementary Table 5 ). These results point to the NTD Q7/Q9 motif that mediates the SG assembly blockade. The Q7/Q9 motif falls within a β-hairpin loop at the NTD that is modulated by the association between CA and cyclophilin [26] . Using the G89A CA mutant that cannot bind CypA, SG assembly was maintained in cells ( Fig. 4c ; Supplementary Table 5 ). Treatment of HIV-1-expressing cells with cyclosporine A (CsA), which mimics the G89A phenotype and effectively disrupts the interaction between CypA and HIV-1 CA [27] , also blocked Gag’s ability to inhibit SG assembly in PatA-treated cells ( Fig. 4d ). Figure 4: Overexposed surface loops in NTD of CA play a crucial role in the inhibition of SG assembly. ( a ) Location of CA amino-acid residues conferring SG dependency are shown in red on the structural model of CA monomer extracted from the hexameric structure (PDB: 3H4E). CA substitutions that did not alter the ability to block SG assembly are shown in green. ( b ) HeLa cells were transfected with five NTD point mutants of CA and exposed to PatA (here Q7A/Q9A). Cells were stained for vRNA, G3BP1 and Gag (p17). Scale bar, 15 μm. ( c ) HeLa cells were transfected with G89A CA mutant or ( d ) WT (pNL4-3) HIV-1 provirus. After 12 h, cells were incubated with 2.5 μM of CsA for 8 h and exposed to PatA. Cells were fixed and stained for vRNA, G3BP1 and Gag (p24). Scale bar, 15 μm. Hela cells were treated with siCypA ( e ) or shCypA ( f ), transfected with WT (pNL4-3) HIV-1 provirus and exposed to PatA. Cells were fixed and stained for G3BP1, TIAR, CypA, vRNA and Gag (p24), as indicated. Scale bar, 10 μm. Red arrows indicate HIV-1-expressing cells. Immunoblot analysis of whole-cell lysates from e , f are shown in right panels. ( g ) Top: CA mutants fail to bind CypA in situ . Nuclei were stained with DAPI (blue), and PLA was performed for Gag and CypA association (red). Bottom: relative quantitation representing spots per cell. Data are represented as mean±s.e.m. Statistical analysis was performed with a one-way analysis of variance (ANOVA) combined with the Bonferroni’s post test. ( h ) Hela cells expressing Gag-GFP were treated with a WT or Q7A/Q9A peptide for 1 h and subjected to PatA. Cells were stained for G3BP1. Scale bar, 15 μm. ( i ) SG present in cells from h were quantified. n =100 cells from three separate experiments. Data are represented as mean±s.d. Full size image To determine the role of CypA in SG assembly, we depleted cellular CypA (also known as PPIA) using either small interfering (si)RNA or short hairpin (sh)RNA lentiviral vectors. Both CypA-targeting approaches depleted CypA to levels achieved previously [28] . The depletion of CypA did not have any effects on SG assembly ( Fig. 4e,f , middle panel). Nevertheless, HIV-1 lost the ability to prevent SG assembly when CypA-depleted cells were subjected to PatA ( Fig. 4e,f , right panel, red arrow). Several studies have shown that the binding of CypA to the CA-exposed loop could shift the position of helix 6, resulting in either the destabilization or repositioning of the β-hairpin at the NTD of CA (residues CA [1] , [2] , [3] , [4] , [5] , [6] , [7] , [8] , [9] , [10] , [11] , [12] , [13] ) where the glutamines at the position 7 and 9 are found [26] , [29] , [30] . To test whether the Q7A/Q9A CA mutant can influence CypA binding, we analysed the association of Gag and CypA using a proximity ligation assay (PLA) that detects protein–protein interactions closer than 40 nm (ref. 31 ). When two proteins interact within a cell, bright fluorescent spots are produced that reveal binding events. The association of Gag wild type (WT) and CypA resulted in an average of 60.31±4.8 spots per cell (s.e.m. ; n =61), whereas the Q7A/Q9A CA-mutant CypA yielded 27.45±2.66 spots per cell ( n =124) and G89A CA-mutant CypA exhibited 18.68±1.77 spots per cell ( n =82). Importantly, only background PLA signals were obtained in the negative control, mock transfected cells (5.8±0.5 spots per cell, n =59) with the calculated differences being highly significant ( Fig. 4g ). These results support the notion that the disruption in the surface-exposed loops of the NTD in newly synthesized HIV-1 CA plays a fundamental role in the Gag-mediated prevention of the stress response. To further explore whether the disruption in the NTD–NTD interface was essential, we synthesized two peptides with an N-terminally conjugated fluorescein isothiocyanate (FITC) group following of the homeodomain of Antennapedia and the first 20 amino acids of CA [32] . Internalization of the CA WT and CA-mutant Q7A/Q9A peptides was measured by FACS as the median fluorescence intensity of HeLa cells that had been treated with one of the FITC-labelled peptides (1–20 μM) for 1 h and then treated with trypsin to degrade cell surface proteins and remove surface ligands, as previously demonstrated [33] . Both WT and Q7A/Q9A peptides were internalized to equivalent extents (data not shown). Gag-GFP-expressing HeLa cells were treated with WT or Q7A/Q9A peptides and subsequently subjected to PatA treatment. Surprisingly, only the treatment with WT peptide led to the assembly of SGs in Gag-expressing cells, while in those treated with the Q7A/Q9A peptide the SG assembly blockade was maintained ( Fig. 4h,i ). Given that both the hexameric and pentameric rings are formed by the NTD–NTD interface of the CA [34] , these results confirm that overexposed loops of the CA NTD are crucial to the block to SG assembly under stress conditions. Gag interacts with eEF2 Several RNAi screens have identified host genes that are involved in practically all steps of HIV-1 replication [35] , [36] , [37] , [38] , [39] , [40] . An independent siRNA screen identified 101 host genes necessary for SG assembly, termed SGDF [6] . Since we demonstrated here that Gag mediates the inhibition of SG assembly, we next identified cellular factors that associate with HIV-1 Gag by liquid chromatography (LC)–mass spectrometry (MS)/MS analysis ( Fig. 5a ). Among the 207 factors with the best scores, four SGDF, eEF2, eukaryotic translation initiation factor 3 subunit 7 (eIF3S7), PRKDC and the 40S ribosomal protein S9 (RPS9) were identified as binding partners of Gag (listed in Supplementary Data 1 ). The results shown in Fig. 1 suggest that inhibition of SG assembly occurs downstream of eIF2α-P, so we focused on eEF2 as a key factor involved in blocking SG assembly in HIV-1-expressing cells. eEF2 is a major player in translation elongation, which catalyses the GTP-dependent translocation of the peptidyl-transfer RNA (tRNA) from the A to P site [14] . Furthermore, the phosphorylation of eEF2 enhances the shut-off of mRNA translation in response to stress [41] . Endogenous eEF2 (eEF2 endo) co-immunoprecipitated weakly with Gag in untreated and stressed cells ( Fig. 5b ). To confirm these results, we created tagged versions of eEF2 that were co-overexpressed with mCherry-Gag (from here on referred as mCh-Gag). mCh-Gag and Flag-eEF2 were co-expressed and immunoprecipitated with anti-Flag or anti-RFP. Reciprocal immunoprecipitations (IPs) showed that mCh-Gag immunoprecipitated with eEF2 and vice versa ( Fig. 5c,d ). We then investigated whether RNA contributes to the interaction between Gag/eEF2, as it does for the Gag/eEF1-α interaction [42] . Cell lysates were mock digested or digested with RNase A before IP. As shown in Fig. 5e , Gag remained associated with eEF2 in the presence of RNase, demonstrating that this interaction is largely RNA independent. Figure 5: Gag interacts with eEF2. ( a ) Flowchart of the proteomics analyses used to define Gag-binding proteins (top). Venn diagram exhibiting the number of overlapping hits between Gag-binding partners with SGDFs (bottom) [6] . ( b ) HeLa cells were transfected with 5 μg of Gag-EGFP or GFP alone and 48 h later were exposed to PatA, lysed and cell extracts were subjected to IP with an anti-GFP antibody. The presence of endogenous eEF2 in the immunoprecipitates was assessed by western blotting. Ten per cent of total cell lysates used in IP are shown as input. ( c , d ) HEK293T cells were co-transfected with mCherry or mCh-Gag and Flag-eEF2 and collected for IP with ( c ) anti-RFP (to detect mCherry ) or ( d ) anti-Flag followed with immunoblot analysis. ( e ) Cell lysates were incubated in the presence (+) or absence (−) of RNase A for 30 min before IP analysis. Data shown are representative of three experiments. ( f ) HeLa cells were transfected with HIV-1 WT (pNL4-3) or CA mutants’ (Q7A/Q9A, G89A) provirus and collected for IP with anti-p24 (to detect Gag ). ( g ) Relative quantitation of eEF2 co-IP with Gag. Ratio of eEF2/Gag for n= 3 experiments. Data are normalized to 1 for Gag WT and represented as mean±s.d. ( h ) Cells from f were subjected to PLA. Nuclei stained with DAPI (blue); PLA performed for Gag and eEF2 (red). Scale bar, 15 μm. ( i ) Relative quantitation of Gag–eEF2 association. Spots per cell were counted. Data represented as mean±s.e.m. of three independent experiments. Statistical analysis was performed with a one-way ANOVA combined with the Bonferroni’s post test. ( j ) HIV-1-expressing HeLa cells were treated with a WT or Q7A/Q9A peptide for 1 h and subjected to PatA. PLA was performed. Top panel: nuclei stained with DAPI (blue); PLA performed for Gag and eEF2 (red). Scale bar, 15 μm. ( k ) Relative quantitation of Gag–eEF2 association. Spots per cell were counted. Data are represented as mean±s.e.m. of three independent experiments. Statistical analysis was performed with a one-way ANOVA combined with the Bonferroni’s post test. ( l ) HEK293T cells were co-transfected with Gag-deletion mutants (MA/CA; MA; CA) fused to Rluc and Flag-eEF2. Cell lysates were IP with anti-RLuc and immunoblotted with anti-Flag (*nonspecific band). Full size image We next examined the ability of CA mutations (in the proviral context) to disrupt the interaction between Gag and eEF2. HEK293T cells were mock transfected or transfected with either HIV-1 WT (pNL4-3; GagWT) or CA-bearing mutant (Q7A/Q9A; G89A) proviral DNAs ( Fig. 5f ). Gag was immunoprecipitated using monoclonal anti-p24 antisera as described in Methods. Endogenous eEF2 co-immunoprecipitated with Gag, confirming our LC–MS/MS data. Nevertheless, co-immunoprecipitated eEF2 tended to be less abundant when we used the Q7A/Q9A or G89A CA mutant ( Fig. 5g ). To confirm this apparent difference in protein interactions, we used PLA as described above ( Fig. 5h ). This approach revealed an astonishing reduction in the Q7A/Q9A–eEF2 ( Fig. 5i , 5.1±0.7 spots per cell, n =38) or G89A–eEF2 ( Fig. 5i , 3.44±0.4 spots per cell, n =49) association in comparison with GagWT-eEF2 ( Fig. 5i , 11.61±2.2 spots per cell, n= 41). Given that Gag-expressing HeLa cells treated with WT peptide led to the assembly of SGs, while in those treated with the Q7A/Q9A peptide the SG assembly blockade was maintained ( Fig. 4h,i ), we used PLA to examine the ability of peptides to modulate the interaction between Gag and eEF2 ( Fig. 5j ). Indeed, the results revealed that HIV-1-expressing cells treated with WT peptide disrupted the Gag–eEF2 interaction by almost 75%, while the treatment with the mutant peptide did not ( Fig. 5k ). These results support our hypothesis that the peptide may interact with the β-hairpin of the CA NTD mimicking the NTD–NTD interface, thereby disrupting the CA–eEF2 interaction. Finally, to show that CA domain is the eEF2-binding determinant, we co-transfected eEF2-Flag and three deletion mutants containing different Gag subdomains (MA/CA, MA and CA) fused in-frame to Rluc (see Fig. 3d ; ref. 20 ) and we performed Co-IP assay using anti-Rluc. The results showed that only MA/CA and CA mutants co-immunoprecipitated with eEF2, while MA did not ( Fig. 5l ). These results confirm the IF analyses shown in the Fig. 3c in which Gag-deletion mutants, that lacked CA, were not able to suppress SG assembly in >70% of transfected cells subjected to PatA ( Supplementary Table 4 ). Taken together, these results define the NTD of Gag, within the CA domain as the region that mediates eEF2 binding. HIV-1 fails to inhibit SG assembly when eEF2 is depleted Since the overexpression and knockdown of many SGDF lead to effects on SG assembly [3] , we evaluated SG assembly in cells transiently transfected with an epitope-tagged version of eEF2. The overexpression of eEF2 was not sufficient to nucleate SGs ( Supplementary Fig. 2a ) and under stress conditions, eEF2 did not localize to SGs, consistent with a previous report [43] . However, the depletion of eEF2 in cells subjected to stress was inhibitory to SG assembly ( Supplementary Fig. 2b,c ; ref. 6 ). Overall, these observations suggest that eEF2 participates in a SG assembly signalling pathway but does not localize to SGs. Next, to confirm that the Gag–eEF2 interaction mediates the inhibition of SG assembly, HIV-1-expressing HeLa cells were treated with sieEF2 followed by treatment with stressors ( Fig. 6a ). In HIV-1-positive cells treated with non-silencing, control siRNA (siNS), SGs were observed in <20% of cells that were subjected to PatA and Ars treatment, as expected ( Fig. 6b , left panel; Fig. 6c , white bar). However, sieEF2 treatment almost completely inhibited HIV-1’s ability to suppress SG assembly, resulting in the appearance of SGs in >70% of HIV-1-positive cells ( Fig. 6b , middle panel; Fig. 6c , grey bar). We rescued eEF2 expression in sieEF2-depleted cells with an eEF2-siRNA-resistant expression construct (Flag-eEF2 R ) and found that the block to SG assembly was restored in HIV-1/Flag-eEF2 R -positive cells ( Fig. 6b , right panel; Fig. 6c , black bar), demonstrating that HIV-1’s capacity to impair SG assembly relies on eEF2 expression. Moreover, the depletion of eEF2 did not affect Gag expression levels ( Fig. 6d,e , white bars) but led to decreased virus production and infectivity to 20% control levels ( Fig. 6e , black and grey bars, respectively). Although the rescue of eEF2 expression by Flag-eEF2 R increased Gag levels, it was not sufficient to revert the defect in virus production. 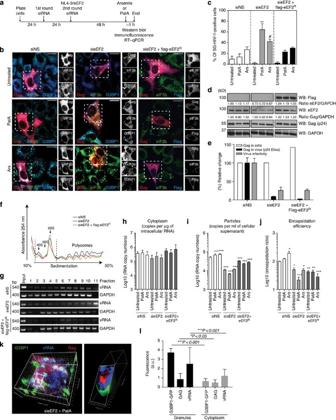Figure 6: Depletion of eEF2 neutralizes Gag. (a) Scheme of the experimental protocol. (b) HeLa cells were treated with siNS (left panel) or sieEF2 (middle panel) and transfected with pNL4-3 or treated with sieEF2 and co-transfected with pNL4-3 and eEF2-siRNA resistant (Flag-eEF2R; right panel). Cells were fixed and stained for G3BP1, eIF3b, Flag (eEF2) and Gag as indicated. Scale bar, 20 μm (c) Quantification of SG in cells fromb. Data are presented as mean±s.d. from three separate experiments with at least 100 cells each analysed. Statistical analysis was performed with a one-way analysis of variance (ANOVA) combined with the Dunnet’s post test (**P<0.01 versus siRNA PatA and#P<0.01 versus siRNA Ars). (d) Cell lysates were analysed for Flag, eEF2, Gag and GAPDH. (e) Effects of depletion of eEF2 on intracellular Gag levels, virus production and infectivity. Graph shows relative change versus siNS-treated cells. Data are presented as mean±s.d. from three separate experiments. (f) HEK293T cells expressing HIV-1 in siNS, sieEF2 or rescue conditions were collected for polysome profile analysis and monitored by continuous ultraviolet absorbance at 254 nm. (g) RNA was isolated in each condition and subjected to RT-PCR. GAPDH mRNA was used as a control. (h) Intracellular vRNA was analysed using quantitative RT–qPCR. Transcript copy numbers per μg of intracellular RNA are shown. (i) Virion-associated RNA was isolated from cell culture supernatants of cells analysed inh. Transcript copy numbers per ml of cellular supernatant were obtained after RT–qPCR analyses. (j) The ratio of virion-associated and intracellular vRNA levels defines the encapsidation efficiency. Data are represented as mean±s.e.m. of three independent experiments. Statistical analysis was performed with a one-way ANOVA combined with the Dunnet’s post test (***P<0.001, **P<0.01, *P<0.05). (k) Left panel: spinning disk confocal microscopy of HIV-1-expressing HeLa cell. Cells were treated with sieEF2 and fixed. G3BP1, Gag and vRNA are identified by FISH/IF. Right panel: insets, 3D reconstruction with cutter edge of the region boxed. (l) Graph shows relative fluorescence intensities of G3BP1, Gag and vRNA within the cytoplasm or G3BP1 granules (n=10 cells). Data are represented as mean±s.d. Statistical analysis was performed with two-way ANOVA combined with the Bonferroni’s post test. Figure 6: Depletion of eEF2 neutralizes Gag. ( a ) Scheme of the experimental protocol. ( b ) HeLa cells were treated with siNS (left panel) or sieEF2 (middle panel) and transfected with pNL4-3 or treated with sieEF2 and co-transfected with pNL4-3 and eEF2-siRNA resistant (Flag-eEF2 R ; right panel). Cells were fixed and stained for G3BP1, eIF3b, Flag (eEF2) and Gag as indicated. Scale bar, 20 μm ( c ) Quantification of SG in cells from b . Data are presented as mean±s.d. from three separate experiments with at least 100 cells each analysed. Statistical analysis was performed with a one-way analysis of variance (ANOVA) combined with the Dunnet’s post test (** P <0.01 versus siRNA PatA and # P <0.01 versus siRNA Ars). ( d ) Cell lysates were analysed for Flag, eEF2, Gag and GAPDH. ( e ) Effects of depletion of eEF2 on intracellular Gag levels, virus production and infectivity. Graph shows relative change versus siNS-treated cells. Data are presented as mean±s.d. from three separate experiments. ( f ) HEK293T cells expressing HIV-1 in siNS, sieEF2 or rescue conditions were collected for polysome profile analysis and monitored by continuous ultraviolet absorbance at 254 nm. ( g ) RNA was isolated in each condition and subjected to RT-PCR. GAPDH mRNA was used as a control. ( h ) Intracellular vRNA was analysed using quantitative RT–qPCR. Transcript copy numbers per μg of intracellular RNA are shown. ( i ) Virion-associated RNA was isolated from cell culture supernatants of cells analysed in h . Transcript copy numbers per ml of cellular supernatant were obtained after RT–qPCR analyses. ( j ) The ratio of virion-associated and intracellular vRNA levels defines the encapsidation efficiency. Data are represented as mean±s.e.m. of three independent experiments. Statistical analysis was performed with a one-way ANOVA combined with the Dunnet’s post test (*** P <0.001, ** P <0.01, * P <0.05). ( k ) Left panel: spinning disk confocal microscopy of HIV-1-expressing HeLa cell. Cells were treated with sieEF2 and fixed. G3BP1, Gag and vRNA are identified by FISH/IF. Right panel: insets, 3D reconstruction with cutter edge of the region boxed. ( l ) Graph shows relative fluorescence intensities of G3BP1, Gag and vRNA within the cytoplasm or G3BP1 granules ( n= 10 cells). Data are represented as mean±s.d. Statistical analysis was performed with two-way ANOVA combined with the Bonferroni’s post test. Full size image To further investigate the involvement of eEF2 in HIV-1 expression, we performed polysome profile analyses ( Fig. 6f ). The depletion of eEF2 slows mRNA translation elongation, which is reflected in the profile as a decrease in the proportion of polysomes and 80S ribosomes ( Fig. 6f , in red). However, the rescue of eEF2 showed a reduction in cellular translation initiation reflected as a decrease in the proportion of polysomes with a concomitant increase in 80S ribosomes ( Fig. 6f , in green). In HIV-1-expressing cells treated with siNS, both vRNA and glyceraldehyde 3-phosphate dehydrogenase (GAPDH) mRNAs were found to be associated with polysomes (see fraction 6–10 in Fig. 6g ). The depletion of eEF2 enhanced vRNA abundance in dense polysome fractions (see fraction 9–11 in Fig. 6g ), while GAPDH was found in monosome fractions (see fraction 3–5 in Fig. 6g ). The rescue of eEF2 produced a shift in the distribution of GAPDH mRNA towards the polysome fractions (see fraction 6–10 in Fig. 6g ), but lead to a shift of vRNA from heavy to light polysomes (see fraction 6–7 in Fig. 6g ). Taken together, these findings indicate that either the depletion or the rescue of eEF2 causes a redistribution of vRNA in polysome profiles that could potentially affect HIV-1’s ability to prevent SG assembly under stress conditions. Reverse transcription–quantitative PCR (RT–qPCR) analyses did not reveal a difference in intracellular vRNA levels when eEF2 was depleted or rescued ( Fig. 6h , compare with siNS). However, vRNA in viral particles ( Fig. 6i ) was found to be decreased 4.6-fold in eEF2-depleted cells possibly reflecting a reduction in vRNA encapsidation while eEF2 expression rescued, albeit incompletely, vRNA levels ( Fig. 6j ). These patterns closely matched the p24 levels in cell-free supernatants ( Fig. 6e , black bars) demonstrating that depletion of eEF2 diminishes the number of viral particles released from cells and the rescue of eEF2 could not completely restore viral production. Given that the levels of intracellular vRNA and Gag expression remain unaffected in eEF2-depleted and rescue cells, we wanted to determine the localization of vRNA in eEF2-depleted cells under stress. 3D reconstruction from spinning disk confocal microscopy images revealed that vRNA was robustly recruited into G3BP1 granules, whereas Gag protein was recruited to a much lesser extent ( Fig. 6k,l ). These results demonstrate that the silencing of eEF2 suppresses virus production and under stress conditions, vRNA/Gag is found sequestered in SGs leading to the loss of Gag’s ability to inhibit SGs. Gag disassembles preformed SGs SG assembly can be triggered by the overexpression of G3BP1 or TIAR [3] . Using this model, we performed IP assays in HEK293T cells overexpressing mCh-Gag, Flag-eEF2 and G3BP1-GFP. The overexpression of G3BP1-GFP interrupted the Gag/eEF2 interaction ( Fig. 7a , lane 6), which was rescued at higher expression levels of Flag-eEF2 ( Fig. 7a , lanes 7 and 8), indicating a possible equilibrium between the association of these two host factors with Gag. In fact, only at low G3BP1-GFP expression levels, the interaction between Gag and eEF2 was preserved ( Fig. 7b , compare lane 5.1). This result was observed over the course of 34 h with G3BP1 being able to displace eEF2 from Gag ( Fig. 7c ). To gain further insight into the specific interaction between Gag and G3BP1, we decided to analyse the dynamics of SG assembly in live cells by inducing SG assembly by G3BP1-GFP overexpression. For this purpose, we co-transfected G3BP1-GFP and mCh-Gag (wild type) and 20 h later examined cells by live cell microscopy (LCM; Fig. 7d ). SG assembly was impaired by the co-expression of mCh-Gag ( Fig. 7e ; Supplementary Movie 1 ; Fig. 1e ) but not when the mCh-GagQ7A/Q9A was co-expressed ( Fig. 7f ; Supplementary Movie 2 ). Moreover, we analysed the association of Gag or GagQ7A/Q9A CA mutant and G3BP1 using the PLA. The association of GagWT and G3BP1 resulted in an average number of 107±19.61 spots per cell ( n =29), whereas that Q7A/Q9A-mutant and G3BP1 showed 33.77±6.4 spots per cell ( n =37; Fig. 7g ). These data validate the role of Gag and the Q × Q motif within the NTD of CA in SG assembly/disassembly. To our surprize, LCM analysis revealed a clearance of preformed SGs that was mediated by Gag expression over time ( Fig. 7h,i ; Supplementary Movie 3 ). Deconvolved optical sections using 3D surface renderings allowed us to visualize how Gag was able to surround G3BP1 structures and begin to dissolve them over time ( Fig. 7i ; Supplementary Movie 3 , inset). Finally, 3D reconstruction of SG foci permitted us to examine the dynamics of SG assembly/disassembly by quantification of the number and size of the SG present within entire cells during the course of the experiment. The quantity and size of SG decreased in the presence of Gag co-expression ( Fig. 7j , black and grey line, respectively). Live cell imaging showed that Gag-mediated SG dynamics fell into two categories: one in which cells expressing G3BP1-GFP did not produce SGs when Gag was expressed and another in which SGs assembled and were maintained for many hours but were dissolved in the presence of Gag. These results indicate that Gag displays a dual role by imposing a blockade to SG assembly and by programming the disassembly of preformed SGs. These data also highlight the importance of translational arrest and SG assembly in the control of HIV-1 infection by innate defences. 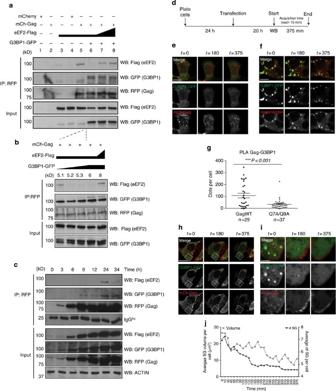Figure 7: G3BP1 overexpression blocks the Gag–eEF2 interaction. (a,b) HEK293T cells were co-transfected with mCh-Gag, Flag-eEF2 and G3BP1-GFP in different concentrations. After 48 h, cells were collected for IP analysis with anti-RFP followed by immunoblot analysis and at different time points (c). Data shown are representative of two independent experiments. (d) Schematic representation of the experimental protocol, including the timing of live cell microscopy (LCM). HeLa cells were co-transfected with G3BP1-GFP and mCh-Gag (e,h) or G3BP1-GFP and mCh-GagQ7A/Q9A (f) and observed under LCM beginning at 20 h post transfection at 15 min intervals. Scale bar, 10 μM (see alsoSupplementary Movies 1 and 2). (g) Cells frome,fwere subjected to PLA. Spots per cell showed the relative quantitation of Gag–G3BP1 (endogenous) association. Data are represented as mean±s.e.m. of three independent experiments. Statistical analysis was performed with a one-way ANOVA combined with the Bonferroni’s post test. (i) Insets represent high-resolution magnification of cell inhwhere SGs disappeared over time of the experiment. Scale bar, 5 μM (see alsoSupplementary Movie 3). (j)Z-stacks were acquired during LCM and imported into IMARIS software. 3D reconstruction was utilized to calculate G3BP1 granule size (volume—grey line). Quantification of SG is shown (#SG—black line). Each data point is the mean collected from four cells analysed. Figure 7: G3BP1 overexpression blocks the Gag–eEF2 interaction. ( a , b ) HEK293T cells were co-transfected with mCh-Gag, Flag-eEF2 and G3BP1-GFP in different concentrations. After 48 h, cells were collected for IP analysis with anti-RFP followed by immunoblot analysis and at different time points ( c ). Data shown are representative of two independent experiments. ( d ) Schematic representation of the experimental protocol, including the timing of live cell microscopy (LCM). HeLa cells were co-transfected with G3BP1-GFP and mCh-Gag ( e , h ) or G3BP1-GFP and mCh-GagQ7A/Q9A ( f ) and observed under LCM beginning at 20 h post transfection at 15 min intervals. Scale bar, 10 μM (see also Supplementary Movies 1 and 2 ). ( g ) Cells from e , f were subjected to PLA. Spots per cell showed the relative quantitation of Gag–G3BP1 (endogenous) association. Data are represented as mean±s.e.m. of three independent experiments. Statistical analysis was performed with a one-way ANOVA combined with the Bonferroni’s post test. ( i ) Insets represent high-resolution magnification of cell in h where SGs disappeared over time of the experiment. Scale bar, 5 μM (see also Supplementary Movie 3 ). ( j ) Z -stacks were acquired during LCM and imported into IMARIS software. 3D reconstruction was utilized to calculate G3BP1 granule size (volume—grey line). Quantification of SG is shown (#SG—black line). Each data point is the mean collected from four cells analysed. Full size image In this work, we demonstrate that HIV-1 evades the translational constraints imposed by both eIF2α-dependent and -independent stresses by subverting host cell machinery that leads to SG assembly. We identified eEF2 as a Gag-associated partner by MS ( Fig. 5 ), a host protein that was also recently found in purified virus [44] . Here, we demonstrate a strict requirement for eEF2 in the Gag-mediated SG assembly blockade. siRNA-mediated depletion of eEF2 not only lead to a defect in the SG blockade imposed by HIV-1 Gag, but also to the sequestration of both Gag and vRNA in SGs, likely leading to the inhibition of viral production ( Fig. 6 ). However, the rescue of eEF2 only restored the Gag-mediated SG blockade but did not restore viral production and infectivity. Given that intracellular vRNA and Gag levels were not markedly affected in both eEF2 depletion or eEF2 rescue conditions, the inability to rescue virus production and infectivity could either be due to the availability of eEF2 for virus assembly or for later functions in reverse transcription complexes, or be due to additional roles for eEF2 in the expression of host factors involved in the assembly/release of HIV-1 particles ( Fig. 6e , Gag in virus; ref. 45 ). Several observations in a mouse model of HIV-1-associated nephropathy revealed a reduction in the phosphorylation of eEF2 resulting in the stimulation of mRNA translation elongation in HIV-1-infected tubular cells [46] . In the ACH-2 cell line, a monocytic model for chronic HIV-1 infection [47] , the activation of eEF2 was triggered concomitantly with the burst in Gag expression during the course of HIV-1 reactivation ( Supplementary Fig. 3 ), suggesting that HIV-1 ensures ongoing viral protein synthesis via enhancing eEF2 activity. While Gag may recruit an eEF2 phosphatase, we propose that Gag impinges on eEF2-P by direct interaction to enhance eEF2 activity to allow for efficient expression of viral proteins and/or cellular proteins that promote virus propagation. Our results also revealed that two glutamines at positions 7 and 9 in the NTD of CA were sufficient to confer the ability of Gag to prevent SG assembly ( Fig. 4 ). When the NTD of CA region is aligned in retroviruses, HIV-1 is the only member possessing the Q × Q motif [24] , suggesting that this motif confers a unique role to this lentivirus’ Gag protein in SG assembly ( Fig. 2 ). Surprisingly, the G89A CA mutant that is defective for CypA binding (a peptidylprolyl isomerase required for optimal HIV-1 infectivity [48] ) and likewise, HIV-1-expressing cells treated with CsA (a drug that impedes the interaction of CypA with HIV-1 CA [49] ), both failed to block SG assembly ( Fig. 4 ). These observations indicate that an interaction between newly synthesized CA and CypA is important to maintain the SG blockade and suggest that CypA may be implicated in the ability of Gag to block the stress response. This notion is supported by the CypA-knockdown experiments, where Gag loses the ability to prevent SG assembly under stress conditions ( Fig. 4 ). Secondary and tertiary structural analyses revealed that in addition to the defined CypA-binding domain in CA (CA 89 ), the N-terminal β-hairpin that precedes helices 1 and 2 in the CA domain folds into an exposed loop [25] ( Fig. 4 ) and currently has no defined host-binding partners. Complete deletion of the NTD does not disrupt particle production, but point mutations interfere with the assembly of the immature CA [34] , suggesting that the interaction of cellular factors in this region would be crucial to HIV-1 replication. Tang et al . [26] showed by NMR that the β-hairpin formation induces a displacement of helix 6 and a subsequent shift of the CypA-binding site. Moreover, the affinity of CypA for Gag is 1,000-fold greater than its affinity for the mature CA protein, suggesting that the β-hairpin- and CypA-binding sites are conformationally coupled [50] . The results obtained with the CA-derived peptide suggest that the interaction with the β-hairpin of Gag might mimic the NTD–NTD interface, thus generating a conformational change in the CypA-binding site and destabilization of the CypA–CA interaction [29] and/or occluding any β-hairpin-binding partner (that is, eEF2), as shown by PLA ( Fig. 5j ). In either of these two scenarios, Gag failed to prevent SG assembly under stress conditions. In this respect, several compounds and peptides that bind to CA have been shown to block early stages of the viral life cycle (reviewed in ref. 51 ). Our results revealed that a CA-derived peptide blocked Gag’s ability to prevent SG assembly presumably by preventing host factor recruitment to newly synthesized HIV-1 CA. Several host proteins (TRIM5α, TNPO3, CPSF6, NUP153, NUP358/RanBP2 and MxB) have been identified as host factors that inhibit HIV-1 infection via interaction with CA (reviewed in ref. 51 ). Whereas these restriction factors are implicated in early HIV-1 replication steps, Manel et al . [52] showed that the interaction between CypA and newly synthesized HIV-1 CA was essential for the innate response to HIV-1 infection in monocyte-derived dendritic cells. In our case, the interaction between eEF2 and newly synthesized HIV-1 CA was indispensable for the prevention of the stress response mounted by the host cell. While HuR, hnRNPA1, hnRNPA2 and TIAR as well as other nuclear proteins shuttle to the cytoplasm and find themselves in SGs during various types of stresses (reviewed in ref. 53 ), HIV-1 did not block nucleocytoplasmic translocation of these SG-resident proteins in infected cells but suppressed their transit into SGs within the cytoplasm (TIAR-GFP; Fig. 1e ). On the basis of our observation that in the absence of eEF2, both vRNA and Gag were recruited to SG, we can infer that Gag targets a late step in SG assembly. In fact, not all RNA granules are made equal and the possibility exists that SG-like granules exist in which translation is active [54] . HIV-1 vRNA is found in Staufen1-containing RNPs [12] as well as in SG-like granules composed of DDX3 and eIF4G [55] . Taken together, these results indicate that Gag inherently prevents SG assembly to disrupt the cellular stress response and that this response might be advantageous for viral replication. We demonstrated, to our surprize, that Gag blocked SG assembly even when G3BP1 and TIAR were overexpressed and effectively dismantled SG induced by G3BP1 ( Supplementary Movie 3 ), suggesting that Gag has far-reaching effects on SG assembly. This relationship was reflected by G3BP1’s ability to inhibit the interaction between Gag and eEF2 in a time-dependent manner ( Fig. 7 ). Therefore, we speculate that the interaction between Gag–eEF2 blocks SG assembly and later, the interaction between Gag–G3BP1 dismantles preformed SG ( Fig. 7 ). Moreover, it would be expected that mRNAs are released from SGs and would be potential substrates for translation. We suspect that the ability of Gag to associate with G3BP1 contributes to the SG blockade by targeting signals that are required for SG assembly, such as the aggregation or phosphorylation status of both G3BP1 and TIAR. The Gag-imposed blockade to SG assembly could confer distinct advantages to HIV-1 under stress conditions. Besides the obvious advantage of maintaining viral mRNA translation, Gag could blunt the deleterious effects of SG assembly when reactive oxygen species (ROS) are induced by viral proteins Nef [56] , Tat [57] and RT [58] . In fact, we showed that Gag expression prevents ROS production under oxidative stress ( Supplementary Fig. 4 ). In addition, Gag expression may prevent the triggering of SG assembly due to a shutdown of translation driven by the HIV-1 protease-mediated cleavage of translation factors [59] . Furthermore, the chronic inflammation and robust production of cytokines and chemokines characteristic of HIV-1 infection in vivo [60] may also lead to massive induction of SGs, a phenomenon that could simply be allayed by the expression of adequate amounts of Gag and Gag/Pol. Remarkably, mRNAs that are translated during stress frequently use non-canonical translational mechanisms [61] . In this scenario, the expression of Gag driven by the activity of the HIV-1 internal ribosome entry site (IRES) at a time when cap- and poly(A)-dependent translation is suppressed would represent an additional means by which HIV-1 secures a replicative advantage [62] . The molecular and cellular details of SG assembly/disassembly may provide clues to prevent and treat degenerative diseases in which SGDF play fundamental roles. Recently, the DYRK3 kinase was found to be a regulator of RNA granules that are formed during cell division and cell differentiation, linking their appearance to the control of mTORC1 signalling [9] . Additional work showed that SGs are cleared by autophagy [10] . In HIV-1-infected macrophages, the viral accessory protein Nef blocks the later stages of autophagosome maturation to allow full Gag processing and increase viral yield [63] . In this context, the sequestration of G3BP1 by Gag could further ensure efficient gene expression and promote HIV-1 biogenesis [12] . A full understanding of the mechanisms governing SG assembly is not yet available, but unravelling how HIV-1 and other viruses affect this process will surely aid in the development of next generation anti-retrovirals [64] . Given the newly defined role for CA in suppressing SG assembly ( Fig. 8 ), a thorough mechanistic understanding may help in the treatment of degenerative diseases where SG proteins contribute to pathology such as in amyotrophic lateral sclerosis, frontotemporal lobar degeneration and spinal motor atrophy, among others [65] , [66] . 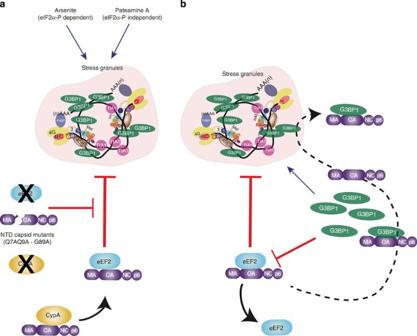Figure 8: Model of Gag in the regulation of SG assembly. (a) The interaction between Gag and eEF2 blocks SG induced by either Ars or PatA. The Gag–CypA association stabilizes the Gag–eEF2 association promoting the block to SG assembly. The depletion of either CypA or eEF2 as well as the expression of CA mutants (Q7A/Q9A; G89A) reverse the phenotype. (b) The overexpression of G3BP1 promotes spontaneous SG assembly. Under this condition, the interaction between Gag and eEF2 blocks SG assembly, but over time, G3BP1 displaces eEF2 from Gag, to promote the disassembly of SG. Figure 8: Model of Gag in the regulation of SG assembly. ( a ) The interaction between Gag and eEF2 blocks SG induced by either Ars or PatA. The Gag–CypA association stabilizes the Gag–eEF2 association promoting the block to SG assembly. The depletion of either CypA or eEF2 as well as the expression of CA mutants (Q7A/Q9A; G89A) reverse the phenotype. ( b ) The overexpression of G3BP1 promotes spontaneous SG assembly. Under this condition, the interaction between Gag and eEF2 blocks SG assembly, but over time, G3BP1 displaces eEF2 from Gag, to promote the disassembly of SG. Full size image Cell culture and transfection conditions HeLa (CCL-2), HEK293T (CRL-11268), NIH3T3 (CRL-1658) and Cos-7 (CRL-1651) cells lines were purchased from the American Type Culture Collection (ATCC). TZM-bl HeLa cell line was obtained from NIH AIDS Reference and Reagent Program. All these cells lines were grown in Dulbecco’s modified Eagle medium (DMEM, Invitrogen) containing 10% fetal bovine serum (FBS, HyClone) and 1% penicillin–streptomycin (Invitrogen). Jurkat (TIB-152, purchased from the ATCC) and ACH-2 cells [47] (obtained from NIH AIDS Reference and Reagent Program) were grown in RPMI 1640 medium (Invitrogen) containing 10% FBS (HyClone) and 1% penicillin–streptomycin (Invitrogen). All cell lines were grown at 37 °C in a 5% CO 2 atmosphere. Cells were transfected with different concentrations of plasmid DNA and/or 20 nM siRNA using Lipofectamine 2000 (Invitrogen) or JetPrime (PolyPlus). HeLa, HEK293T, NIH3T3 and Cos-7 cells were collected 48 h later unless otherwise indicated. Jurkat T cells were collected at day 6 post transfection. ACH-2 cells were induced with 2 ng ml −1 phorbol 12-myristate 13-acetate (Sigma-Aldrich) for 1 h. Medium was replaced and cells were collected at time points up to 72 h. For imaging studies, HeLa, NIH3T3 and Cos-7 cells were seeded onto sterile coverslips, and for Jurkat T, PBMC and ACH-2 cells, sterile poly- L -lysine-coated (Sigma-Aldrich) coverslips were dropped into wells and cells were allowed to settle onto these for 4 h before stress induction and fixing with 4% paraformaldehyde (EMD Millipore). Samples from HIV-1-infected subjects We studied PBMC samples from two HIV-1-infected subjects and one uninfected healthy donor. Frozen and thawed PBMCs from the HIV-infected subjects were obtained from leukophoresis samples. The long-term nonprogressor subjects were from the Canadian Cohort of HIV-infected slow progressors and the typical progressor was from the Québec Primary Infection Cohort. Supplementary Table 1 provides information on the clinical characteristics of these subjects. The PBMC sample from the uninfected healthy donor was isolated by density-gradient centrifugation (Ficoll-Paque, Pharmacia, Upsala, Sweden) from whole blood obtained by venipuncture into tubes containing EDTA anticoagulant. All subjects provided informed consent for participating in this study. The research ethics boards of the recruiting sites, the Centre Hospitalier de l’Université de Montréal and the Véritas Institutional Review Board as well as the site where experiments with human cells were done, McGill University Health Centre, approved this study. Stress induction and drug treatment To induce stress, PatA (from Jerry Pelletier, McGill University, Canada) and sodium Ars (NaAsO 2 ; Sigma-Aldrich) were used. PatA was diluted in media to a final concentration of 300 nM and applied to cells for 1 h before collection. Ars was diluted to a final concentration of 0.5 mM and applied to the cells for 45 min before collection. CsA (Calbiochem) was diluted to a final concentration of 2 μM and the treatment was performed 8 h post transfection. Plasmids The proviral DNA constructs used were: pNL4-3 (an HIV-1 proviral clone expressing the full complement of viral proteins); HIV-2 GFP (a vector based on pSVR, an infectious proviral clone of HIV-2 ROD containing a simian virus 40 origin of replication and a deletion in ENV, which was replaced by CMV-GFP, was provided by Andrew Lever (University of Cambridge, UK)); MLV (a full-length infectious proviral clone) was provided by Guy Lemay (Université de Montréal, Canada); SIV (a full-length infectious proviral clone, SIVmac239/WT) was provided by Chen Liang (McGill University, Canada); RSV (a clone containing the RSV Schmidt-Ruppin subgroup proviral genome lacking v-src, with the pol gene replaced by that of the RSV Bryan high-titer strain) was provided by Volker Vogt (Cornell University, USA); FIV (an FIV gag-pol expression vector deleted for Env, Vif, LTRs and the FIV RNA packaging signal, pFP93) was provided by Eric Poeschla (Mayo Clinic, USA); EIAV (a Gag-Pol vector pONY3.1, an GFP-packaging vector pONY8.0 and pMD-G, which encodes the envelope glycoprotein of the vesicular stomatitis virus were used to produce pseudotyped EIAVGFP virus) was provided by Lionel Berthoux (UQTR, Canada); pNL4-3vif(−), pNL4-3vpr(–), pNL4-3vpu(–), pNL4-3env(–) and pNL4-3nef(–) were provided by Klaus Strebel (NIAID, NIH). SVBH10(myr−), proviral clone based on BH10 with the genotype vif−, vpr 72AA , vpu −, and nef −, which contains a mutation in Vpr and does not possess the Gag-MA myristoylation signal, was kindly provided by Lawrence Kleiman (McGill University, Canada); HxBruΔP6, proviral clone that lacks of the vpu and nef viral genes and contains a deletion of Gag-domain p6, was kindly provided by Heinrich Gottlinger (University of Massachusetts, USA); pTat(−)GV/4GS was kindly provided by the late Teh Jeang (NIH, USA) and contains a full-length HXB2 proviral HIV-1 genome, in which a termination codon replaces the ATG (methionine) initiation codon in the Tat-coding region. The resulting mutant is unable to synthesize Tat. This clone contains four copies of Gal4-binding sites inserted in both the 5′ and 3′ LTR and a Gal4-VP16 gene inserted in-frame in nef allows efficient LTR transactivation in the absence of Tat; pMRev(−), proviral clone that introduces a termination codon in place of the glycine residue 6 (GGA) in the rev gene and a leucine (CTG) codon in place of arginine (CGG) at residue 52 of the tat reading frame. The resulting mutant is unable to synthesize Rev, but expresses functionally intact and active Tat; pVRC4200 and pVRC4000 Gag,Gag/Pol expression constructs were kindly provided by Lawrence Kleiman (McGill University, Canada); pNLXX, proviral clone that contains a six-nucleotide mutation that produces an amber nonsense codon (TAG) in place of the gag initiation codon and a nonsense mutation within CA (residue 109, residue 241 of Pr55 Gag ), was provided by David Ott (National Cancer Institute, NCI, USA). Gag-mutant plasmids used were Gag/Rluc, MA/CA-Rluc, MA-Rluc, CA-Rluc and p2-p1-Rluc. All MA-deleted mini-Gag proviruses (MAΔ36-57, MAΔ36-87, MAΔ8-87, MAΔ8-126 and MAΔ1-126) were provided by Heinrich Göttlinger (University of Massachussetts, USA). All proviral point mutants in the CA domain (Q7A/Q9A, R18A/N21A, E28A/E29A, P38A, A42D and G89A) were donated by Chris Aiken (Vanderbilt University, USA). CA-deletion mutants (CAΔ1-48, CAΔ61-148, CAΔ61-148, CAΔ149-193 and CAΔ194-231) were generated using pCMV-GagM1-10 as template (provided by George Pavlakis, Centre for Cancer Research, USA). pGag-EGFP was obtained from NIH AIDS Reference and Reagent Program. To generate CA-EGFP, CA domains was recovered from pNL4-3 using primers 5′- GCTCGAGCCCCTATAGTGCAGAACCTC -3′ and 5′- CGGGATCCCAAAACTCTTGCTTTATGGC -3′. The amplicon was digested with XhoI and BamHI and inserted in pEGFP-C1(Clontech). mCherry and mCh-Gag were provided by Paul Bieniasz (Rockefeller University, USA). mCh-GagQ7A/Q9A and CAQ7AQ9A-EGFP were performed by QuickChange Site-Directed Mutagenesis Kit (Stratagene) according to the manufacturer. Gag-mapping constructs were made using template GagM1-10. PCR products were made with specific deletions and then ligated into the construct using SalI and BamHI. G3BP1-GFP was provided by Imed Gallouzi (McGill University, Canada). TIAR-GFP was provided by Ricardo Soto-Rifo (ICBM, Chile). eEF2 cDNA was obtained from OpenBiosystem and cloned in pcDNA3.1-Myc/His (Invitrogen) between XbaI and HindIII or pCI-Neo-Flag (Invitrogen) between XhoI and NotI. Flag-eEF2 from mouse was kindly provided by Yi-Shuian Huang (Academia Sinica, Taiwan). pEGFP-C1 (Clontech) and pcDNA3.1 DNA (Invitrogen) were included in transfection mixes to supplement total amounts of DNA or were always supplemented in control transfections. RNA interference and antibodies Non-silencing control siRNA and siRNAs targeting eEF2#1 (5′- CCGCGCCATCATGGACAAGAA -3′), eEF2#2 (5′- CGCCCTCTTAGTAGGGACTTA -3′) and PPIA/CypA (5′- CTGGGTGATACATTCAATGT -3′) were purchased from QIAGEN-Xeragon. shRNA DNA clones that target CypA (shCypA1, TRCN0000049228) and the shRNA that contains the scrambled target sequence were purchased from Sigma-Aldrich. Mouse anti-p24 (1:400), rabbit anti-p24 (1:400), sheep anti-p17 (1:400) and SIV anti-gp120 (1:400) were obtained from the NIH AIDS Reference and Reagent Program. MLV anti-p30 (1:400) was from National Cancer Institute/Biological Carcinogenesis Branch Repository (USA); RSV anti-CA (1:400) was generously provided by Volker Vogt (Cornell University, USA); FIV anti-CA (1:400) was generously provided by Eric Poeschla (Mayo Clinic, USA); anti-UPF1 (1:200) was generously provided by Jens Lykke-Anderson (University of California-San Diego, USA); anti-G3BP1 (1:10,000), anti-TIAR-1 (1:500), anti-eIF3b (1:250) and anti-His (1:400) were purchased from Santa-Cruz Biotechnology; anti-ACTIN (1:10,000), anti-eIF2α (1:1,000), anti-eIF2α-P (1:1,000) and anti-eEF2 (1:2,000) were purchased from Abcam; anti-eEF2 (1:2,000) and anti-eEF2-P (1:2,000) were from Cell Signaling; anti-Rluc (1:1,000) was obtained from Sigma and MBL; anti-GFP (1:10,000) and sheep anti-digoxin (1:250) were from Roche; anti-Flag (1:2,000), anti-PABP (1:200) and mouse anti-digoxin (1:400) were from Sigma-Aldrich; anti-GAPDH (1:2,500) was purchased from Techni-Science; anti-RFP (1:2,000) was purchased from Allele Biotechnology; anti-Myc (1:2,000) from US Biological; anti-HRP secondary conjugated antibodies were purchased from Rockland Immunochemicals (1:5,000); and AlexaFluor secondary antibodies and 4′,6-diamidino-2-phenylindole (DAPI) were from Life Technologies (1:500). Western blotting For immunoblot analyses, cells were collected after transfection, washed with PBS (Life Technologies) and lysed in lysis buffer (100 mM NaCl, 10 mM Tris, pH 7.5, 1 mM EDTA, 0.5% Nonidet P-40, protease and phosphatase inhibitor cocktail (Roche) and RNase Out (Life Technologies)). Cell lysates were quantified by the Bradford assay (Bio-Rad), and equal quantities of protein were loaded into SDS–PAGE gels. Proteins were then transferred onto nitrocellulose membranes (Bio-Rad Laboratories) and blocked with 10% defatted milk (Carnation) in Tris-buffered saline (TBS), 0.1% Tween-20. Blocked membranes were first incubated with primary antibodies of interest and then with secondary antibodies conjugated to horseradish peroxidase (Rockland Immunochemicals). Signals were exposed by autoradiography following development with Western Lightning Chemiluminescence Reagents as described by the manufacturer (Perkin-Elmer). Proteins were quantified on film using the ImageJ software (NIH: http://rsbweb.nih.gov/ij/index.html ). Scans of the most important blots are shown in Supplementary Fig. 5 . Fluorescence in situ hybridization, immunofluorescence and imaging analyses FISH/IF co-analyses have been described in detail elsewhere [67] . In brief, after transfection, cells were washed once in PBS (Invitrogen) and fixed with 4% paraformaldehyde (EMD Millipore) for 20 min. Cells were then washed with PBS, incubated in 0.1 M glycine for 10 min, washed with PBS, incubated in 0.2% Triton X-100 (Merck) for 5 min, washed in PBS and stored in 70% ethanol at 4 °C. A digoxigenin-labeled RNA probe was synthesized in vitro in presence of digoxigenin-labeled UTP (Roche). To stain the vRNA, cells were rehydrated in PBS and DNAse (Invitrogen) treated for 15 min (25 U per coverslip), then incubated in hybridization solution for 16–18 h at 42 °C (50% formamide, 1 mg ml −1 tRNA, 2 × SSPE, 5 × Denharts, 5 U RNaseOut, 50 ng probe). Cells were then incubated in 50% formamide for 15 min at 42 °C and incubated twice in 2 × SSPE for 5 min each at 42 °C. Cells were briefly washed in PBS before being blocked in 1 × blocking solution (Roche). Primary antibodies were applied for 1 h at 37 °C, and then washed for 10 min in PBS followed by secondary antibodies for 1 h. Cells were washed for 20 min in PBS before being mounted on glass slides using ImmunoMount (Thermo Fisher Scientific). Laser confocal microscopy was performed using a Leica DM16000B microscope. The microscope was equipped with a WaveFX spinning disk confocal head (Quorum Technologies, Ontario, Canada), and images were acquired with a Hamamatsu ImageEM EM-charge-coupled device camera. Signals from images obtained with AlexaFluor 647 were pseudocoloured in blue. Scanning was performed and digitized at a resolution 1,024 × 1,024 pixel. Filter sets and laser wavelengths were described earlier [18] , [68] . All imaging experiments were performed at least three times with similar results. Imaging analyses were performed by Imaris software v. 7.6 (Bitplane). AutoDeblur software (Autoquant X2; Media Cybernetics) was used for deconvolution. The observed phenotypes were representative of n >100 cells per condition in each experiment. SGs were defined as large G3BP1 foci measuring >0.5 μm (ref. 8 ). Live cell microscopy Cells were plated onto four-well Lab-Tek II-covered chamber slides at 50% confluency. Before imaging, media were replaced with phenol-red-free DMEM with 25 mM HEPES (Invitrogen) and 10% FBS. Slides were incubated in a live-cell-imaging humidified chamber that was maintained at 37 °C and 5% CO 2 . LCM was performed using a Leica DM16000B microscope described above. Volocity Imaging software (v4.3.2; Perkin-Elmer) was used as acquisition software. 3D reconstruction analyses were performed by Imaris software v. 7.6 (Bitplane). The excitation for GFP was 491 nm and the filter was 525/50 nm. The excitation for mCherry was 561 nm and the filter was 595/50 nm. Infectivity assay Virion-containing supernatants were clarified by centrifugation at 2,000 g for 10 min at 4 °C followed by filtration (0.2 μm). Virus collected from supernatants was quantified using the HIV-1 p24 Capture ELISA kit (Advanced BioScience Laboratories). TZM-bl HeLa cells were infected and 24 h later, cells were lysed in passive lysis buffer and luciferase activity was measured by Dual-Luciferase Reporter Assay System according to the manufacturer’s directions (Promega). Viral infectivity was determined by dividing luciferase activity by virus concentration (p24 levels, ELISA assay). vRNA encapsidation assay and RT–qPCR Determination of intracellular and virion-associated RNA copy numbers of transfected HEK293T cells was done as follows. Forty-eight hours post transfection, the medium was collected and centrifuged for 5 min at 300 g and 4 °C. Cell-free supernatants were filtered through a 0.45-μm filter and ultracentrifuged at 35,000 g for 1 h at 4 °C. Pellet was resuspended in 80 μl of lysis buffer described above. Fifteen μl of concentrated particles was used for western blot analysis, while 65 μl was used to do vRNA extraction using TRIzol-LS Reagent according to the manufacturer’s instructions (Invitrogen). HEK293T cells were washed in cold PBS (Invitrogen) and cytoplasmic fractions were lysed in lysis buffer described above. Nuclei were pelleted by centrifugation for 2 min at 300 g and 4 °C followed by careful collection of the supernatant as cytoplasmic fraction. Subsequently, the TRIzol-LS reagent was used to extract cytoplasmic RNA according to the manufacturer’s instructions (Invitrogen). For quantitative RT–PCR, total RNA was reverse transcribed using Super Script II (Invitrogen) and then used for quantitative PCR analysis with specific primers for unspliced viral RNA (genomic RNA) forward 5′- TACAGGAGCAGATGATACAG -3′ and reverse 5′- CCTGGCTTTAATTTTACTGG -3′. All RT–qPCR reactions were performed with SsoFAST Evagreen supermix (Bio-Rad) and a 7500 Fast Real-Time PCR system (Applied Biosystems). Copy numbers per μg of intracellular vRNA or per ml of analysed cell culture supernatants were calculated and mean values of log10-transformed copy numbers are reported. Control reactions without RT were also performed regularly and demonstrated the successful removal of transfected plasmid DNA by the DNase treatment (Life Technologies). Peptide synthesis The chimeric peptide consisting of Antennapedia domain (RQIKIWFQNRRMKWKK) and the first 20 amino acids of CA was synthesized at the McGill Peptide Synthesis Laboratory (PTI Sonata). The peptides were purified to 85% purity and analysed using HPLC. Two peptides were synthesized; one containing the WT sequence of the first 20 amino acids of CA and a mutant containing glutamine (Q) to alanine (A) mutations at the 7th and 9th positions of CA. The peptides were dissolved in UltraPure DNase/RNase-Free Distilled Water (Invitrogen) at a concentration of 1 mM. To perform the internalization assay, new peptides with an N-terminally conjugated FITC group were synthesized by Tenova Pharmaceuticals and their purities (99%) were assessed by analytical HPLC. Internalization of the peptide WT and MUT (Q7A/Q9A) was measured as the median fluorescence intensity of HeLa cells that had been treated with one of the FITC-labelled peptides (1–20 μM) at 37 °C for 1 h, and then treated with trypsin to degrade cell surface proteins and remove surface ligands. In situ PLA assays In situ PLA detection was carried out using the DUOLINK II In Situ kit obtained from OLINK Bioscience (Uppsala, Sweden) according to the protocol of the manufacturer. In brief, cells were subjected to blocking using the DUOLINK blocking solution (1 drop) at 37 °C for 30 min. Primary antibodies were added at a dilution of 1:50 in 40 μl DUOLINK antibody diluent and incubated at 37 °C for 1 h. The slides were washed two times with wash buffer A for 5 min each, then secondary antibodies (DUOLINK anti-rabbit PLA-plus probe, DUOLINK anti-mouse PLA-minus probe) were added and incubated at 37 °C for 1 h. Two washes with wash buffer A were then followed by addition of the ligation mix and incubation at 37 °C for 30 min, followed by another two washes. Thereafter, the amplification reaction was carried out at 37 °C for 100 min. Subsequently, the slides were washed twice with wash buffer B and once with 0.1 × wash buffer B. Mounting was done with DuIn Situ Mounting Medium with DAPI. Images were acquired using a Leica DM16000B microscope. The microscope was equipped with a WaveFX spinning disk confocal head (Quorum Technologies, Ontario, Canada), and images were acquired with a Hamamatsu ImageEM EM-charge-coupled device camera. Corresponding TIF files were then used for quantification using BlobFinder (Version 3.2). PLA signals were detected as local maxima applying a 3 × 3 pixel mask. Nuclei had to have a minimum diameter of 100 pixels for detection [69] . IP assays HeLa and HEK293T cells were transfected as described above. Briefly, 1 mg of protein was immunoprecipitated with agarose-conjugated anti-GFP beads for 2 h as described by the manufacturer (MLB). For red fluorescent protein (RFP) IP, 1 mg of protein was immunoprecipitated with magnetic anti-RFP beads for 2 h as described by the manufacturer (MLB). For p24 IP, 1 mg of protein was pre-cleared with normal mouse or rabbit serum and 25 μl of a 50:50 slurry of protein A-Sepharose or protein G-Sepharose (Thermo Scientific), incubated with mouse (NIH AIDS Reference and Reagent Program) or rabbit (Fritzgerald) anti-p24 (American BioTechnologies; dilution 1:200) for 16 h at 4 °C and with 30 μl of 50:50 slurry of protein A-Sepharose or protein G-Sepharose for 2 h at 4 °C. For Rluc IP, 1 mg of protein was incubated with rabbit anti-Rluc (MBL) for 16 h at 4 °C, and with 30 μl of 50:50 slurry of protein A-Sepharose for 2 h at 4 °C. The bound complexes were analysed by SDS–PAGE analysis [70] . LC–tandem MS analysis HeLa cells were transfected with Gag-GFP and 48 h later, cells were collected. GFP was immunoprecipitated by using agarose-conjugated anti-GFP beads as described by the manufacturer (MBL). The proteins eluted were separated on 4–15% SDS–PAGE (Bio-Rad) and the bands excized and analysed by LC–MS/MS at SAMS Centre for proteomics, University of Calgary. Gel slices were cut into 1 mm 2 pieces and rinsed once with 200 μl HPLC grade water, then twice with 200 μl of 50 mM ammonium bicarbonate in 50% acetonitrile. Gel pieces were dried in a speedvac, then rehydrated in 12.5 ng μl −1 trypsin solution in 25 mM ammonium bicarbonate pH 8. Once gels were hydrated with trypsin solution, 25 mM ammonium bicarbonate was added to cover gel (~10–20 μl) and samples were kept at 37 °C overnight. Extraction of peptides from gel pieces was done twice with 50 μl 1% formic acid in 50% acetonitrile and supernatant pooled. Samples were dried down and reconstituted in mobile phase A for injection into LC system. Digests were analysed using a Thermo Orbitrap Velos. Injected samples were first trapped and desalted on a Acclaim pepmap trap column (3 μm, 2 cm × 75 μm inside diameter; Dionex) for 4 min with 3% acetonitrile/0.2% formic acid delivered at 4 μl min −1 . The peptides were then reverse eluted from the trapping column and separated on an analytical Acclaim Pepmap (2 μm, 15 cm × 75 μm inside diameter; Dionex) at 0.3 μl min −1 . Data-dependent acquisition of collision-induced dissociation MS/MS was utilized, and parent ion scans were run over the mass range m / z 300–1,750. For analysis of LC–MS/MS data, Mascot searches used the following parameters: 10 p.p.m. MS error, 0.8 Da MS/MS error, one potential missed cleavage and variable oxidation (Met). FACS analysis For apoptosis assays, HeLa cells were transfected as described above and 24 h later were treated with Annexin V (Invitrogen) and DAPI (Sigma-Aldrich) staining according to the manufacturer’s instructions (Invitrogen). Etoposide (1 μM, Sigma) was used as positive control. For the ROS assay, HeLa cells were transfected as described above and 24 h later were treated for CellROX staining according to the manufacturer’s instructions (Invitrogen). Stained cells were analysed on a flow cytometer (LSRFortessa; BD Biosciences). H 2 O 2 (50 nM) was used as positive control. Assays were performed in duplicate for each sample. Phylogenetic analysis Sequences were retrieved from the GenBank database. A phylogenetic tree with 500 bootstrap replicates was constructed with the neighbour-joining method using MEGA 6.0 software. Statistical analysis The statistical data analysis and graphics described in the text were done using the GraphPad v6.0 program (La Jolla, CA, USA). Differences were tested by unpaired two-tailed Student’s t -test or analysis of variance (Dunnet’s or Bonferroni’s post test) where P <0.05 was considered significant. How to cite this article: Valiente-Echeverría, F. et al . eEF2 and Ras-GAP SH3 domain-binding protein (G3BP1) modulate stress granule assembly during HIV-1 infection. Nat. Commun. 5:4819 doi: 10.1038/ncomms5819 (2014).